A NIGT1-centred transcriptional cascade regulates nitrate signalling and incorporates phosphorus starvation signals inArabidopsis Nitrate is a nutrient signal that triggers complex regulation of transcriptional networks to modulate nutrient-dependent growth and development in plants. This includes time- and nitrate concentration-dependent regulation of nitrate-related gene expression. However, the underlying mechanisms remain poorly understood. Here we identify NIGT1 transcriptional repressors as negative regulators of the Arabidopsis NRT2 . 1 nitrate transporter gene, and show antagonistic regulation by NLP primary transcription factors for nitrate signalling and the NLP-NIGT1 transcriptional cascade-mediated repression. This antagonistic regulation provides a resolution to the complexity of nitrate-induced transcriptional regulations. Genome-wide analysis reveals that this mechanism is applicable to NRT2 . 1 and other genes involved in nitrate assimilation, hormone biosynthesis and transcription. Furthermore, the PHR1 master regulator of the phosphorus-starvation response also directly promotes expression of NIGT1 family genes, leading to reductions in nitrate uptake. NIGT1 repressors thus act in two transcriptional cascades, forming a direct link between phosphorus and nitrogen nutritional regulation. Nitrogen (N) is a key plant macronutrient that is a major constituent of abundant essential compounds such as amino acids, nucleotides and chlorophyll [1] . N availability therefore has a profound effect on plant growth and productivity [1] , [2] . In order to thrive, plants adapt to fluctuations and differences in N availability in their environments through modulation of gene expression and metabolism. Nitrate in soils is the major N source for plants. Unlike microorganisms that use nitrate as an N source only in the absence of preferred energy-effective N sources such as ammonium and glutamine, higher plants take up and use nitrate to synthesise N-containing compounds even in the presence of other N sources [3] . Consistent with this preference, nitrate also serves as a signalling molecule that induces a variety of nitrate responses in plants [4] , [5] . Modulation of plant gene expression by nitrate is complex. Nitrate provision immediately induces the expression of a wide variety of genes, including nitrate transport- and assimilation-associated genes, genes involved in phytohormone synthesis and response, and genes encoding regulatory proteins such as transcription factors and protein kinases [6] , [7] . Recent studies with Arabidopsis provide critical insights into the molecular mechanisms underlying nitrate-responsive gene expression. NIN-LIKE PROTEIN (NLP) transcriptional activators, which are highly conserved in plants, act as the primary transcription factors controlling the nitrate response [8] , [9] . Nitrate triggers Ca 2+ signalling and activates calcium sensor kinases CPK10, CPK30 and CPK32. The CPKs phosphorylate NLPs at a conserved serine residue, and then phosphorylated NLPs accumulate in the nucleus and activate target genes [10] . The primary event in nitrate-induced transcriptional regulation is thus post-translational. Although the physiological functions of only two of the nine Arabidopsis NLPs (NLP7 and NLP8) are known, most NLPs are thought to be involved in the nitrate response [8] , [9] , [11] , [12] , [13] , [14] . Several additional transcription factor genes are induced by nitrate, and the encoded transcription factors are thought to evoke secondary transcriptional responses that activate or repress a new set of genes. Accordingly, these transcription factors produce a broad range of outcomes or modulate the expression of NLP targets by positive or negative feedforward mechanisms [15] , [16] , [17] , [18] . Although NLPs are known to directly regulate several nitrate-inducible genes through binding at specific cis -elements in the 5′ or 3′ flanking regions of the genes [9] , [14] , [19] , [20] , [21] , and nitrate-inducible transcription factors are known to be involved in the nitrate response [15] , [16] , [18] , transcriptional cascades involving NLPs have not been characterised. Thus, the molecular mechanisms underlying the complex regulation of gene expression during the nitrate response remain to be elucidated. Arabidopsis NRT2 . 1 , a typical nitrate-inducible gene, encodes a major high-affinity nitrate transporter that is indispensable for vigorous plant growth under nitrate concentrations in the natural ecosystem [22] , [23] . NRT2 . 1 expression is rapidly and strongly induced upon provision of nitrate to N-starved or ammonium-cultivated Arabidopsis plants [24] . Upregulation is transient, and is suppressed within a few hours, suggesting that a time-dependent regulatory mechanism is also active [24] . Nitrate concentration also controls the steady-state levels of NRT2 . 1 expression. Nitrate is most effective in promoting NRT2 . 1 expression at low concentrations, with high concentrations (>0.5 mM) curbing the effect [24] , [25] , [26] . Similar responses were also reported for barley and Nicotiana plumbaginifolia NRT2 genes [27] , [28] . Several factors participating in the regulation of NRT2 expression were identified. For example, NLP7 binding at the NRT2 . 1 promoter enhanced the expression [9] , TCP20 transcription factor also bound to the NRT2 . 1 promoter [29] , and HNI9/AtIWS1 repressed expression of Arabidopsis NRT2 . 1 under high N conditions through trimethylation of histone H3 [30] . However, although the complex regulation of NRT2 expression underpins its role in managing nitrate uptake in natural conditions [31] , the transcriptional repressor that modulates NRT2 expression in a time- and nitrate concentration-dependent manner remains to be identified. Many other nitrate-inducible genes are also regulated in a time-dependent manner [16] , [32] , [33] , suggesting that an unknown regulatory mechanism might orchestrate the synchronous expression of these genes. However, such a mechanism is completely unknown. Group II genes of the LBD gene family in Arabidopsis ( LBD37-39 ) are potential negative regulators involved in time- and nitrate concentration-dependent modulations of nitrate-inducible gene expression [17] . LBD37-39 are nitrate-inducible, and enhanced and reduced expression of several N metabolism-associated genes is seen with loss-of-function mutants and overexpression lines, respectively [17] . Another negative regulator candidate is NITRATE-INDUCIBLE GARP-TYPE TRANSCRIPTIONAL REPRESSOR1 (NIGT1). Rice NIGT1 ( Os NIGT1) is a nitrate-inducible gene-encoded transcriptional repressor that binds to 5′-GAATC-3′ and 5′-GAATATTC-3′ [16] , [34] . With the exception of Os NIGT1 targeting of Os NIGT1 for negative feedback regulation, targets of Os NIGT1 remain to be identified; however, transgenic rice overexpressing Os NIGT1 exhibits nitrate response-related phenotypes [16] . Arabidopsis possesses four homologues of Os NIGT1. The homologues of Os NIGT1 and three additional proteins with relatively lower similarities comprise the HRS/HHO family in Arabidopsis [35] , [36] . Although involvement of Arabidopsis homologues of Os NIGT1 in the phosphorus (P)-starvation response was suggested [35] , [36] , [37] , they are candidates for negative regulators for nitrate response due to their very strong induction by nitrate [7] , [36] . Intriguingly, N uptake was reduced by P limitation in several plant species [38] , [39] , [40] , probably to maintain the balance of N and P metabolism. In the light of the suggested involvement of Arabidopsis Os NIGT1 homologues in P-starvation response, they are also candidates for the regulators causing downregulation of nitrate uptake under P-starvation conditions. To reveal the molecular mechanisms underlying complex regulation of gene expression during the nitrate response, we identify transcriptional repressors of the NRT2 . 1 promoter in this study. The NRT2 . 1 promoter is suppressed by Arabidopsis NIGT1 homologues, which are encoded by direct target genes of NLPs. Furthermore, expression of these genes is directly enhanced by the PHOSPHATE STARVATION RESPONSE 1 (PHR1) master regulator of P-starvation response [41] , [42] , inducing P-starvation-induced downregulation of nitrate uptake. These findings uncover two transcriptional cascades that govern complex expression of nitrate-inducible genes and for integration of N and P signalling. NIGT1.1 is a negative regulator of NRT2 . 1 Expression of NRT2 . 1 is immediately repressed after activation in nitrate-treated Arabidopsis seedlings, suggesting that a transcriptional repressor might control repression. Scrutinisation of the NRT2 . 1 promoter sequence revealed that it includes consensus sequences for NIGT1- (5′-GAATC-3′) and LBD-binding (5′-GCGGCG-3′) [43] (Fig. 1a , Supplementary Fig. 1 ). To examine whether Arabidopsis homologues of Os NIGT1 and LBDs were negative regulators of NRT2 . 1 , a reporter plasmid harbouring the luciferase reporter gene ( LUC ) under the control of the NRT2 . 1 promoter was co-transfected into protoplasts alongside an effector plasmid for expression of LBD37 or an Arabidopsis homologue of Os NIGT1 (NIGT1.1). Protoplasts were prepared from N-starved Arabidopsis plants to allow detection of nitrate-responsive activation of the NRT2 . 1 promoter caused by endogenous NLPs [20] . Nitrate-induced activation was detected when an empty vector was used as a control effector plasmid, and NLP7 expression enhanced nitrate-responsive activation of the NRT2 . 1 promoter as reported previously [9] (Fig. 1b ). Nitrate-dependent activation and NLP7-induced enhancement were both suppressed by co-expression of NIGT1.1, whereas co-expression of LBD37 had almost no impact on NRT2 . 1 promoter activity. This indicated that NIGT1.1 had a specific negative effect on the NRT2 . 1 promoter and also that NIGT1 could override the NLP7-driven activation of NRT2 . 1 expression in response to nitrate (Fig. 1b ). Fig. 1 Repression of the NRT2 . 1 promoter by NIGT1.1. a Structure of the NRT2 . 1 promoter. Consensus sequences for NIGT1 binding (5′-GAATC-3′) and LBD binding (5′-GCGGCG-3′) are indicated by red and green bars, respectively. White and black boxes indicate the 5′ untranslated and coding regions, respectively. Probe DNAs used in EMSA ( c , d ) are shown below the promoter structure. To disrupt the NIGT1-binding sequences, mutated probes contained nucleotide substitutions, indicated by X. b Activation of the NRT2 . 1 promoter by nitrate and NLP7 and repression by NIGT1.1 in protoplasts. Protoplasts co-transfected with the NLP7, NIGT1.1 or LBD37 expression vector or the empty vector (none) together with the reporter plasmid containing the LUC gene fused to the NRT2 . 1 promoter were incubated in the presence of 1 mM KCl or KNO 3 . In b and e , LUC activity was normalised with GUS activity from the reference UBQ10-GUS plasmid and data are means ± s.d. of three biological replicates. c , d EMSA with recombinant NIGT1.1 protein and DNA probes from the NRT2 . 1 promoter. Red arrowheads indicate positions of protein–DNA complexes caused by binding of NIGT1.1 to probe DNA. The Os NIGT1 probe served as a positive control. e Effects of disruption of the NIGT1-binding sites on the NRT2 . 1 promoter activity in protoplasts. Protoplasts co-transfected with the LUC gene fused to the wild-type or mutant NRT2 . 1 promoter and the NLP7 expression vector or an empty vector were incubated in the presence of 1 mM KCl or KNO 3 . X indicates disrupted NIGT1 sites. f ChIP analysis of the NRT2 . 1 promoter using Col and NIGT1.1-OX seedlings. Four regions were amplified by PCR with immunoprecipitated DNA. Data are means of four biological replicates with s.d. ** p < 0.01 by one-tailed t test. g Effects of disruption of the NIGT1-binding sites on NRT2 . 1 promoter activity in the presence of abundant N. Five seedlings of transgenic lines harbouring the LUC gene fused to the wild-type [ NRT2 . 1p (WT)- LUC ] or the mutated [(mut1+2)-LUC] NRT2 . 1 promoter were incubated with (+) or without (−) 10 mM NH 4 NO 3 for 24 h. Images of LUC activity in vivo and bright-field images were captured in two independent transgenic lines. Bar, 2 cm Full size image To examine the role of Arabidopsis NIGT1s in controlling NRT2 . 1 expression, NIGT1-binding sites in the NRT2 . 1 promoter were investigated using an electrophoretic mobility shift assay (EMSA) with recombinant NIGT1.1 protein (Fig. 1c, d ). NIGT1.1 bound specifically to probe p5 (−217 to +63, relative to the transcription start site) (Fig. 1c ), which contained three copies of the putative NIGT1 site (Fig. 1a ), and we therefore examined the effects of mutations in these sites (conversion of 5′-GAATC-3′ to 5′-tAcTC-3′). The results indicated that NIGT1.1 bound to the first and second sites in the proximal region of the NRT2 . 1 promoter but not to the third one (Fig. 1d ). Consistent results were obtained in co-transfection experiments with reporter plasmids containing LUC under the control of mutated NRT2 . 1 promoters harbouring the same mutations (Fig. 1e ). Simultaneous disruptions of the first and second GAATC sequences significantly abolished NIGT1.1-dependent repression (Fig. 1e ), while disruptions of the third one did not affect NIGT1.1-dependent repression (Supplementary Fig. 2 ). Thus, NIGT1.1 repressed the NRT2 . 1 promoter through interactions at these two sites. Any mutations on the NIGT1-binding sites did not affect NLP7-induced activation of the NRT2 . 1 promoter (Fig. 1e , Supplementary Fig. 2 ). We therefore hypothesised that NLP7 and NIGT1.1 independently regulated the NRT2 . 1 promoter. To confirm this, we identified NLP-binding sites in the NRT2 . 1 promoter. We sought for putative NLP-binding sites in two regions homologous between the NRT2 . 1 and NRT2 . 2 promoter sequences, because NRT2 . 2 , another high-affinity nitrate transporter gene neigbouring NRT2 . 1 , very resembles NRT2 . 1 in both expression pattern and structure [22] , [44] . Since two putative NLP-binding sites (−714 to −707 and −172 to −150) were found in the homologous regions (Supplementary Fig. 1 ), EMSA were performed with DNA probes containing these sites. Consequently, NLP7 was shown to bind to both sites (Supplementary Fig. 3a,b ). Co-transfection assays consistently indicated that the disruption of either site reduced NLP7-dependent transactivation and also that the disruption of both sites almost diminished both nitrate-inducible activation and NLP7-dependent transactivation (Supplementary Fig. 3c−e ). Furthermore, the disruption of these sites did not affect the NIGT1.1-induced repression (Supplementary Fig. 3f ), indicating that NLP7 and NIGT1.1 independently regulate the NRT2 . 1 promoter through interactions with distinct sites. The binding of NIGT1.1 to the NRT2 . 1 promoter in planta was also corroborated using transgenic Arabidopsis plants overexpressing MYC-tagged NIGT1.1 (NIGT1.1-OX lines) (Supplementary Fig. 4 ). Chromatin immunoprecipitation (ChIP) analysis using the NIGT1.1-OX line revealed that NIGT1.1 specifically bound to the proximal promoter region containing the identified NIGT1-binding sites (Fig. 1f ). NIGT1-binding site-dependent repression of the NRT2 . 1 promoter was further characterised using in vivo imaging of LUC activity. We introduced LUC under the control of wild-type and mutated NRT2 . 1 promoters into the wild-type Arabidopsis and examined LUC activity in seedlings of the obtained transgenic lines (Fig. 1g ). LUC production decreased upon N supplementation (ammonium nitrate) with both wild-type and mutated promoters, but the decrease was far weaker with the mutated promoter, indicating that NIGT1 binding at these sites was associated with repression of NRT2 . 1 promoter activity. In vivo imaging also clarified concentration-dependent nitrate induction of the NRT2 . 1 promoter and also suggested that NIGT1-mediated repression is evident in the presence of high concentrations of nitrate (Supplementary Fig. 5 ). Together, these results indicate that NIGT1.1 acts as a negative regulator of NRT2 . 1 and competes with positive regulation by NLPs. Redundancies of NIGT1 - clade genes in Arabidopsis Phylogenic analysis indicated a particularly close relationship between Os NIGT1 and four Arabidopsis proteins of the HRS/HHO family [17] , [37] , [38] as demonstrated by very high bootstrap values (Fig. 2a ). Os NIGT1 and these four proteins were distinguishable from others of the HRS/HHO family and formed a separate clade [16] , [35] , [36] , referred to hereafter as the NIGT1 clade (Fig. 2a ). Previous microarray analysis showed that all of the Arabidopsis NIGT1-clade genes ( NIGT1 . 1/HHO3 , NIGT1 . 2/HHO2 , NIGT1 . 3/HHO1 and NIGT1 . 4/HRS1 ) were induced by nitrate treatment [7] . We therefore examined whether these genes exhibited similar expression patterns and whether their roles were redundant. RT-quantitative real-time PCR (qPCR) analysis was used to characterise the temporal and nitrate concentration-dependent expression of these genes (Fig. 2b, c ). Nitrate treatment of nitrate-starved seedlings induced expression of NIGT1-clade genes; however, no induction was seen with ammonium, glutamine or trans -zeatin (tZ), a type of cytokinin (N response-related phytohormone) (Fig. 2d ). These expression patterns were similar to those of Os NIGT1 [16] and NRT2 . 1 . This suggested that all NIGT1-clade genes were primary nitrate-inducible genes, like NRT2 . 1 . However, NIGT1 . 1 and NIGT1 . 2 induction was less pronounced than induction of NIGT1 . 3 and NIGT1 . 4 (Fig. 2b−d ), and NIGT1 . 1 and NIGT1 . 2 were expressed in both shoots and roots in contrast with the root-specific expression of NIGT1 . 3 and NIGT1 . 4 (Supplementary Fig. 6a ). Fig. 2 NIGT1 proteins redundantly regulate NRT2 . 1 expression. a Phylogenic analysis of Arabidopsis and rice NIGT1/HHO proteins. Arabidopsis and rice proteins are shown in black and blue, respectively. Numbers indicate bootstrap values of 1000 iterations. b Time-dependent expression patterns of NIGT1-clade genes after 10 mM KNO 3 supply. c Concentration-dependent induction by nitrate. RNA was prepared from ammonium-grown seedlings before treatment and after treatment with 0, 0.1, 0.5, 1 and 10 mM KNO 3 for 1 h. A 10 mM KCl treatment was used as a control. d Nitrate-specific induction of NIGT1 - clade genes. Ammonium-grown seedlings were treated for 1 h with 10 mM of each chemical, except for trans- zeatin (5 µM). e Repression of the NRT2 . 1 promoter by NIGT1 proteins. Protoplasts co-transfected with NIGT1 expression vectors or the empty vector (none) together with the reporter plasmid containing the LUC gene under the control of the NRT2 . 1 promoter were incubated in the presence of 1 mM KCl or KNO 3 . LUC activity was normalised to GUS activity from the co-transfected UBQ10-GUS plasmid. Data are means ± s.d. of three biological replicates. f Transcript levels of NRT2 . 1 in the nigt1 quadruple mutants ( Q-1 and Q-2 ) and NIGT1.1-OX plants after 10 mM KNO 3 supply. Values are normalised to those of UBQ10 , and are means of biological triplicates ± s.d. ( b , c , d , f ) Full size image NLPs direct the majority of primary nitrate-induced gene expression [8] , [9] . Our transcriptome analysis with transgenic Arabidopsis in which NLP activity was reduced by the expression of a chimera repressor NLP6-SUPRD (NLP6-SUPRD lines) [21] also suggested that nitrate-inducible expression of NIGT1-clade genes was under the control of NLP activity [21] . We thus performed co-transfection assays to examine whether NLP7 activated the promoters of NIGT1-clade genes (Supplementary Fig. 7 ). The 1 kb promoters of NIGT1 . 1 , NIGT1 . 3 and NIGT1 . 4 were activated by co-expression of NLP7 in the presence of nitrate, suggesting the existence of the NLP-NIGT1 transcriptional cascade. Neither nitrate- nor NLP7-dependent activation of the NIGT1 . 2 promoter was observed in this assay, suggesting that nitrate-responsive cis -elements for NIGT1 . 2 may be outside the promoter fragment used. Co-transfection experiments also showed that all Arabidopsis NIGT1s were transcriptional repressors of the NRT2 . 1 promoter (Fig. 2e ). This suggests that Arabidopsis NIGT1s have a redundant role in regulating NRT2 . 1 expression. Time-course analysis of expression of the NIGT1-clade genes suggested that NLP-NIGT1 transcriptional cascade-mediated suppression of NRT2 . 1 occurred after activation by NLPs. This antagonistic relationship may be involved in downregulation of NRT2 . 1 expression after a transient peak induced by nitrate treatment. We therefore analysed the time-dependent expression pattern of NRT2 . 1 in nigt1 . 1 nigt1 . 2 nigt1 . 3 nigt1 . 4 quadruple mutants ( nigtQ-1 and Q-2 ) and NIGT1.1-OX lines (Fig. 2f ). A transient NRT2 . 1 expression peak was observed in all lines, but expression levels were higher in the quadruple mutants and lower in the two independent NIGT1.1-OX lines. Furthermore, modified levels of NRT2 . 1 transcripts in the single, double, triple and quadruple nigt1 mutants suggested that all NIGT1 -clade genes are involved in the regulation of NRT2 . 1 expression (Supplementary Fig. 8c ), consistent with the expression of NIGT1-clade genes in outer cell layers in roots (Supplementary Fig. 6c ) where NRT2 . 1 is expressed [25] , [26] , [45] . The relatively higher expression level of NIGT1 . 4 in cortex and root hair-forming cells [35] (Supplementary Fig. 6b ) might correlate with the stronger effect of the nigt1 . 4 mutation on NRT2 . 1 expression (Supplementary Fig. 8c ). Genome-wide survey of target genes of the NLP-NIGT1 cascade Time-dependent expression control after nitrate supply is not specific to NRT2 genes but is common to many nitrate-inducible genes [16] , [32] , [33] . To investigate whether antagonistic regulation by NLP and the NLP-NIGT1 cascade modulated the expression of other genes, a genome-wide survey of the target genes of the NLP-NIGT1 cascade was performed using previous transcriptome data of nitrate-responsive genes [7] and genes that were downregulated in Arabidopsis NIGT1.2 overexpressors (accession number GSE100903 in Gene Expression Omnibus) [46] (Fig. 3 , Supplementary Data 1 and 2 ). The combined survey revealed that out of 1343 genes induced by nitrate after 30 min or 3 h [7] , 271 genes (20%) were repressed by constitutive overexpression of NIGT1.2 (Fig. 3a ). Lower expression levels of these genes in the NLP6-SUPRD lines [21] were confirmed, suggesting that these genes are under the control of NLP activity (Supplementary Data 1 ). Therefore, these genes are likely under the control of both NLP-mediated activation and NLP-NIGT1 transcriptional cascade-mediated repression, and expression of these genes may thereby transiently increase after nitrate supply. The gene list includes not only N transport and assimilation-associated genes ( NRT2 . 1 , NRT2 . 2 , NAR2 . 1 , etc. ), but also genes involved in iron metabolism, the oxidative pentose phosphate (OPP) pathway for supplying reducing power for N assimilation, transcription ( TGA1 [15] and HYH ), and hormone metabolism ( IPT3 , CYP735A2 [47] , TAR2 , and CYP707A2 , 3 [14] ) (Fig. 3a , Supplementary Data 1 ). Like NRT2 . 1 , NAR2 . 1 (also called NRT3 . 1 ), which encodes an accessory protein essential for NRT2.1 activity [45] , [48] , exhibited a time-dependent expression pattern that was modulated in nigtQ mutants and NIGT1.1-OX lines (Fig. 4a ). Furthermore, ChIP assay with the NIGT1.1-OX line suggested that NIGT1 bound specifically to a region of the NAR2 . 1 promoter that contained consensus sequences for NIGT1 binding (Fig. 4b ). This suggests that the molecular mechanism consisting of nitrate signalling, NLPs, and the NIGT1 transcriptional cascade coordinately modulates expression of NRT2 . 1 and NAR2 . 1 to control nitrate uptake activity in response to the abundance of environmental nitrate. CYP735A2 and HYH were also identified as possible targets of NLPs and the NLP-NIGT1 cascade (Fig. 3a ). CYP735A2 encodes cytokinin hydroxylase, which catalyses the biosynthesis of tZ-type cytokinin, and HYH encodes a bZIP transcription factor involved in light-mediated development. Expression of these genes was similarly downregulated in NIGT1.1-OX plants, and NIGT1.1 specifically bound to the regions of their promoters containing NIGT1-recognition sequences in vivo (Supplementary Fig. 9 ). Hence, antagonistic regulation by NLPs and the NLP-NIGT1 cascade likely modulates the expression of a variety of genes associated with the nitrate response. For further investigation of physiological relevance of the NLP-NIGT1 cascade, we focused on CYP735A2 , because this gene encodes a key enzyme for biosynthesis of tZ-type cytokinin that is intimately associated with nitrate response [47] , [49] . We measured the tZ content in the NLP6-SUPRD line, the nlp6 nlp7-1 double mutant, the nigt1 quadruple mutant, and the NIGT1.2 overexpressor line (Fig. 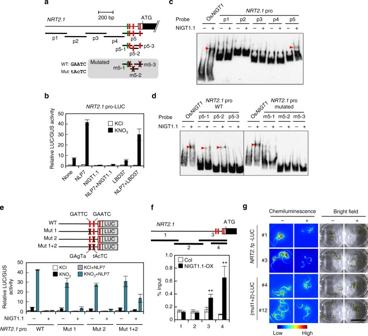Fig. 1 Repression of theNRT2.1promoter by NIGT1.1.aStructure of theNRT2.1promoter. Consensus sequences for NIGT1 binding (5′-GAATC-3′) and LBD binding (5′-GCGGCG-3′) are indicated by red and green bars, respectively. White and black boxes indicate the 5′ untranslated and coding regions, respectively. Probe DNAs used in EMSA (c,d) are shown below the promoter structure. To disrupt the NIGT1-binding sequences, mutated probes contained nucleotide substitutions, indicated by X.bActivation of theNRT2.1promoter by nitrate and NLP7 and repression by NIGT1.1 in protoplasts. Protoplasts co-transfected with the NLP7, NIGT1.1 or LBD37 expression vector or the empty vector (none) together with the reporter plasmid containing theLUCgene fused to theNRT2.1promoter were incubated in the presence of 1 mM KCl or KNO3. Inbande, LUC activity was normalised with GUS activity from the reference UBQ10-GUS plasmid and data are means ± s.d. of three biological replicates.c,dEMSA with recombinant NIGT1.1 protein and DNA probes from theNRT2.1promoter. Red arrowheads indicate positions of protein–DNA complexes caused by binding of NIGT1.1 to probe DNA. The OsNIGT1probe served as a positive control.eEffects of disruption of the NIGT1-binding sites on theNRT2.1promoter activity in protoplasts. Protoplasts co-transfected with theLUCgene fused to the wild-type or mutantNRT2.1promoter and the NLP7 expression vector or an empty vector were incubated in the presence of 1 mM KCl or KNO3. X indicates disrupted NIGT1 sites.fChIP analysis of theNRT2.1promoter using Col and NIGT1.1-OX seedlings. Four regions were amplified by PCR with immunoprecipitated DNA. Data are means of four biological replicates with s.d. **p< 0.01 by one-tailedttest.gEffects of disruption of the NIGT1-binding sites onNRT2.1promoter activity in the presence of abundant N. Five seedlings of transgenic lines harbouring theLUCgene fused to the wild-type [NRT2.1p(WT)-LUC] or the mutated [(mut1+2)-LUC]NRT2.1promoter were incubated with (+) or without (−) 10 mM NH4NO3for 24 h. Images of LUC activity in vivo and bright-field images were captured in two independent transgenic lines. Bar, 2 cm 5 , Supplementary Table 1 ). Supply of nitrate strongly increased the tZ content in the N-starved wild-type seedlings, and this increase was impaired in the NLP6-SUPRD and nlp6 nlp7-1 lines. On the other hand, the quadruple nigt1 mutation enhanced the nitrate-induced increase in the tZ content, whereas the overexpression of NIGT1.2 alleviated it. These results revealed a role of NIGT1 proteins in modulating the NLP-mediated physiological response. Fig. 3 Nitrate-responsive and NIGT1-regulated genes. a A Venn diagrams showing an overlap between genes upregulated by nitrate after 30 min or 3 h and genes downregulated in NIGT1.2-overexpressing plants. b A Venn diagram showing an overlap between genes downregulated by nitrate after 30 min or 3 h and downregulated in NIGT1.2-overexpressing plants. Numbers of genes are shown. Note that NRT2 . 4 was upregulated at 30 min after nitrate treatment but downregulated at 3 h Full size image Fig. 4 Repression of NAR2 . 1 by NIGT1s. a Time-dependent expression of NAR2 . 1 in Arabidopsis Col, nigt1 quadruple mutants ( Q-1 and Q-2 ), and two NIGT1.1-OX lines (#9 and #15). Seedlings were harvested at the indicated time points after supply of 10 mM KNO 3 . Values are normalised with expression levels of UBQ10 , and means of biological triplicates ± s.d. are shown. b Binding of NIGT1.1 to the NAR2 . 1 promoter in vivo. ChIP analysis was carried out with Col and NIGT1.1-OX seedlings. Two different regions of the NAR2 . 1 promoter that contained or did not contain putative NIGT1-recognition sequences (red bars) were amplified from immunoprecipitated DNA by PCR. Data are means of four biological replicates with s.d. ** p < 0.01 by one-tailed t -test compared with corresponding values obtained with Col seedlings Full size image Fig. 5 NLP and NIGT1 activity affects tZ-type cytokinin content. Cytokinin contents in the seedlings treated with 1 mM KNO 3 or KCl for 24 h were measured. The cytokinin contents in two NLP6-SUPRD lines were compared with those in its parental line (4xNRE-35Smin-GUS) [21] , and the cytokinin contents in the nlp6 nlp7-1 mutant, the nigt1 quadruple mutant ( nigtQ-3 ), and the complementation line of nigtQ-3 , which was produced by expression of NIGT1 . 2 , were compared with those in Col seedlings. The cytokinin contents in the NIGT1 overexpressor (NIGT1.2-GFP-OX), which was produced by the overexpression of NIGT1.2 fused to GFP, were compared with those in the GFP overexpressor line (GFP-OX). Values are mean ± s.d. ( n = 4~5). Different letters denote significant difference by Tukey’s HSD ( p < 0.05) Full size image Our genome-wide survey also provided a list of genes whose expression was reduced by both nitrate treatment and NIGT1 overexpression (Fig. 3b , Supplementary Data 2 ). These genes appear to be regulated by the NLP-NIGT1 cascade alone, and thereby they are candidates for the genes whose expression is negatively regulated by nitrate signalling. Of 1126 genes downregulated by nitrate treatment, 260 genes were downregulated in the NIGT1.2 overexpressor, including genes encoding transporters for nitrate, ammonium and ureide, and transcription factors. Autoregulation of NIGT1-clade genes Our genome-wide survey suggested that NIGT1-clade genes might themselves be targets of the NLP-NIGT1 cascade (Fig. 3a ). This is consistent with the previous evidence suggesting that OsNIGT1 is autoregulated [16] . Co-transfection assays were used to determine whether NIGT1-clade genes in Arabidopsis were autoregulated (Fig. 6a ). NIGT1.1 suppressed the promoters of all the NIGT1-clade genes. Furthermore, in transgenic Arabidopsis plants constitutively overexpressing NIGT1.1, NIGT1 . 2-1 . 4 and endogenous NIGT1 . 1 exhibited reduced levels of time-dependent gene expression in both the presence and absence of nitrate (Fig. 6b ). In a ChIP assay using the NIGT1.1-OX line, regions that contained putative NIGT1-binding sites conserved in Arabidopsis NIGT1 - clade genes and Os NIGT1 , but not in other HHO genes [16] (regions 2, 4, 6 and 8), specifically co-immunoprecipitated with NIGT1.1, suggesting that NIGT1s bound specifically to these conserved sites in vivo (Fig. 6c ). Co-expression of NIGT1.1 also decreased both nitrate-induced activation and NLP-dependent transactivation of the NIGT1 . 1 and NIGT1 . 3 promoters (Fig. 6d ). These results suggest that feedback regulation of NIGT1-clade genes is mediated by NIGT1 transcriptional repressors, indicating that nitrate signalling is complex and is driven by the integration of the NLP-NIGT1 cascade and the NIGT1 autoregulation. Fig. 6 Autoregulation of NIGT1-clade genes. a Repression of NIGT1-clade gene promoters by NIGT1.1. A reporter plasmid that contained the LUC gene under the control of an NIGT1 promoter was co-transfected in protoplasts alongside the NIGT1.1 expression vector and the UBQ10-GUS reference plasmid. LUC activity was normalised with GUS activity. Data are means ± s.d. of three biological replicates. b Reduced expression of endogenous NIGT1 . 1 as well as NIGT1 . 2 , NIGT1 . 3 and NIGT1 . 4 in NIGT1.1-OX lines. Ammonium-grown Arabidopsis Col and NIGT1.1-OX seedlings were treated with 10 mM KNO 3 for the indicated periods and used for RT-qPCR analysis. Values are normalised to UBQ10 expression levels, and means of biological triplicates with s.d. are shown. c Binding of NIGT1.1 to the NIGT1 gene promoters in vivo. ChIP analysis was performed with Col and NIGT1.1-OX seedlings. Two different promoter regions were amplified from immunoprecipitated DNA. Data are means of four biological replicates with s.d. ** p < 0.01 by one-tailed t test compared with corresponding values obtained with Col seedlings. Positions of the conserved and nonconserved putative NIGT1-binding sites are shown by vertical red and orange lines, respectively. d Antagonistic regulation of NIGT1-clade gene promoters by NLP7 and NIGT1.1. Expression vectors for NLP7 and NIGT1.1 were co-transfected into protoplasts at different ratios, together with a reporter plasmid containing the LUC gene under the control of the NIGT1 . 1 or NIGT1 . 3 promoter. Transfected protoplasts were incubated in the presence of 10 mM KCl or KNO 3 . LUC activity was normalised with GUS activity, and relative LUC activities are means ± s.d. of three biological replicates Full size image PHR1 activates the promoters of NIGT1-clade genes Nitrate uptake is repressed by P starvation [38] , [39] , [50] . Although expression of NIGT1 - clade genes is strongly induced by nitrate, several previous studies suggested that the NIGT1-clade genes might also be involved in the P-starvation response [35] , [36] , [37] . Supporting this, DNA microarray data provided previously by Bustos et al. [42] suggested that expression of NIGT1 . 1 , 1 . 2 and 1 . 3 likely decreased in an Arabidopsis phr1 phl1 mutant. PHR1 and its close homologue, PHR1-LIKE1 (PHL1), are key transcriptional activators that recognise the 5′-GNATATNC-3′ sequence (called P1BS) [41] and orchestrate P-starvation-induced gene expression [42] . PHR1, PHL1 and NIGT1s belong to the GARP family of plant transcription factors, and the P1BS sequence overlaps with one of the NIGT1-recognition sequences (5′-GAATATTC-3′) [16] , [34] . Thus, we hypothesised that PHR1 and PHL1 might directly activate expression of NIGT1-clade genes through binding to NIGT1-binding sites and other P1BS sites to downregulate NRT2 . 1 expression. To test this hypothesis, we initially confirmed the effects of P starvation and phr1 phl1 double mutation on the expression of NIGT1 - clade genes using RT-qPCR analysis. P starvation upregulated the expression of all NIGT1-clade genes, and this upregulation was compromised in the phr1 phl1 mutant (Fig. 7a ). NRT2 . 1 expression was strongly downregulated under the P-starved conditions, but downregulation was alleviated in phr1 phl1 . Furthermore, co-transfection assays with the PHR1 expression vector revealed that PHR1 activated the NIGT1 . 1 , NIGT1 . 2 and NIGT1 . 3 (but not NIGT1 . 4 ) promoters in vivo (Fig. 7b ). Next, the sites mediating PHR1-dependent transactivation in the NIGT1 . 1 promoter were determined using mutational analysis. Three copies of P1BS are found within the NIGT1 . 1 promoter, one of which is also a conserved NIGT1-binding site (Fig. 7c ) [16] . The disruption of each P1BS slightly decreased activation by PHR1 (Supplementary Fig. 10 ). Simultaneous disruption of all three copies of P1BS reduced the promoter activity by half compared with the wild-type promoter (Fig. 7c , Supplementary Fig. 10 ). Unexpectedly, disruption of the proximal NIGT1-binding sequence (5′-GATTC-3′) also reduced promoter activity to half that of the wild-type promoter (Fig. 7c ), and the simultaneous disruption of this GATTC sequence and all three copies of P1BS mostly abolished activation by PHR1 (Fig. 7c ), indicating that these sites were recognised by PHR1. Co-transfection assays also revealed that, as with the combination of NLP7 and NIGT1s, transactivation caused by PHR1 was suppressed by co-expression of NIGT1s, indicating competition between PHR1-dependent activation and NIGT1-dependent repression on the expression of NIGT1-clade genes in vivo (Fig. 7d ). Furthermore, ChIP assays with transgenic Arabidopsis plants overexpressing PHR1 suggested that PHR1 bound to the proximal region of the NIGT1 . 1 promoter and other NIGT1-clade gene promoters in vivo (Fig. 7e ). Slight amplification of regions 1, 3, 5 and 7 was probably because sonication in the ChIP procedure causes inhomogeneous fragmentation of DNA. These results indicated the existence of the PHR1-NIGT1 transcriptional cascade. Although the identified PHR1-binding sites in proximal regions were conserved in all NIGT1 promoters, the recovery of the corresponding region of the NIGT1 . 4 promoter (region 8) was lower than in other NIGT1-clade gene promoters (regions 2, 4 and 6) and very similar to the value of a region not containing P1BS (region 7) in the ChIP assays. This was consistent with relatively lower induction of NIGT1 . 4 expression and no transactivation of the NIGT1 . 4 promoter by PHR1. Because not all P1BS motifs are functional for P-starvation response [42] , the sequences surrounding the P1BS motif in the NIGT1 . 4 promoter might affect its functionality. Fig. 7 PHR1-dependent activation of NIGT1-clade genes. a Effects of P starvation on the expression of NIGT1-clade genes and NRT2 . 1 in roots of Arabidopsis Col and phr1 phl1 double mutant. Roots of Arabidopsis plants that were grown hydroponically under P-sufficient (+P) or P-starved (−P) conditions for 5 days were used for RT-qPCR analysis. IPS1 is a positive control for P starvation. Values are normalised with expression levels of PEX4 , and means of biological triplicates with s.d. are shown. * p < 0.05, ** p < 0.01 by two-tailed t -test compared with corresponding Col values. b Transactivation of NIGT1 promoters by PHR1. A reporter plasmid containing 1 kb promoter fragments of NIGT1 - clade genes fused to the LUC gene was co-transfected into protoplasts with the PHR1 expression vector or an empty vector (none) and the UBQ10-GUS plasmid. c Identification of sites mediating PHR1 regulation and autoregulation in the NIGT1 . 1 promoter. Transactivation of wild-type and mutated NIGT1 . 1 promoters by PHR1 and repression by NIGT1.1 were analysed by co-transfection assays. The horizontal line indicates the 1 kb NIGT1 . 1 promoter. Vertical black and red lines indicate the P1BS sequences and the conserved NIGT1 sites, respectively. Mutated sites are indicated with blue X. d Competitive regulation of the NIGT1-clade gene promoters by PHR1 and NIGT1. Expression vectors for PHR1 and NIGT1.1 were co-transfected into protoplasts at different ratios, together with the LUC reporter gene under the control of the NIGT1 . 1 or NIGT1 . 3 promoter. In b − d , relative LUC activity is given as mean ± s.d. of three biological replicates. e Binding of PHR1 to the NIGT1-clade gene promoters in vivo. Two different regions from each NIGT1-clade gene promoter were amplified in a ChIP assay of transgenic plants expressing MYC-tagged PHR1 cultured under the P-starved condition. The IPS1 promoter is a known target of PHR1 and is used as a positive control, and PP2A is a negative control. Data are means of three biological samples and shown with s.d. * p < 0.05, ** p < 0.01 by one-tailed paired t -test compared with corresponding control (no antibody) values Full size image The role of the PHR1-NIGT1 cascade in nitrate uptake PHR1-NIGT1 cascade-dependent regulation of the NRT2 . 1 promoter activity was investigated by in vivo imaging of LUC activity in transgenic plants harbouring LUC fused to the wild-type promoter or a mutant promoter with disrupted NIGT1-binding sites [mut(1+2) promoter in Fig. 1e ]. Levels of LUC activity driven by the wild-type and mutant NRT2 . 1 promoters were similar under the P-sufficient condition, and LUC levels decreased in both after P-starvation treatment for 3 days. However, LUC levels were higher with the mutant than with the wild type under P-deficient conditions (Fig. 8a ), indicating that NIGT1-binding sites were partly involved in P-starvation-induced repression of the NRT2 . 1 promoter. Because NRT2.1 is the high-affinity nitrate transporter that plays the major role in uptake of nitrate from soils, we next examined nitrate uptake activity of wild-type plants and nigt1 quadruple mutants grown with or without P (Fig. 8b ). Nitrate uptake was comparable between wild-type plants and nigt1 quadruple mutants under the P-sufficient condition. Nitrate uptake decreased in P-starved seedlings, but uptake was higher in the nigt1 quadruple mutant than in the wild type under the P-deficient condition (Fig. 8b ). These results suggest that P starvation partly influences nitrate uptake through the PHR1-NIGT1-NRT2.1 transcriptional cascade. Fig. 8 The PHR1-NIGT1 cascade modulates nitrate uptake. a NIGT1-binding site-mediated P-starvation response of NRT2 . 1 promoter activity. Transgenic Arabidopsis seedlings harbouring the LUC gene under the control of the wild-type or (mut1+2) mutant NRT2 . 1 promoter were grown under P-sufficient (+P) or P-starved (−P) conditions for 3 days and then treated with 1 mM luciferin. Images of LUC activity in living seedlings were captured in two independent transgenic lines. Scale bar, 1 cm. b Nitrate uptake activity of nigt1 quadruple mutants ( Q-1 and Q-2 ) during P starvation. 15 NO 3 − uptake by Arabidopsis Col and mutant seedlings grown hydroponically under P-sufficient (+P) or P-starved (−P) conditions for 5 days was measured at 0.2 mM K 15 NO 3 . Values are means of five biological replicates ± s.d. ** p < 0.01 by two-tailed t -test Full size image In the current study, we identified the NLP-NIGT1 and PHR1-NIGT cascades, both of which downregulate NRT2 . 1 in opposition to direct activation by NLPs. These findings demonstrate the molecular mechanisms underlying the complex regulation of the expression of nitrate-inducible genes. The identification of the NLP-NIGT1 cascade allows us to propose a simple model to explain the transiently high expression and subsequent downregulation that are very frequently exhibited by primary nitrate-inducible genes after nitrate treatment (Fig. 9a ). In this model, nitrate-activated NLPs at first rapidly maximise the expression levels of their targets and then expression is downregulated by NLP-induced NIGT1s. Thus, the transcript levels of these genes are determined by the balance of activated forms of NLPs and NIGT1s. Although we demonstrated antagonistic regulation by NLP7 and NIGT1s only at the NRT2 . 1 promoter, the same mechanism likely applies to downregulation of other nitrate-inducible genes, including N metabolism- and hormone-related genes and transcription factor genes for the secondary nitrate response (Fig. 3 ). In fact, we showed that nitrate-induced increases in the cytokinin content were modified under the control of NLP and NIGT1 activities (Fig. 5 , Supplementary Table 1 ). Hence, NIGT1 proteins act as modulators for nitrate-responsive transcription, and the antagonistic regulation by NLPs and the NLP-NIGT1 cascade may be critical to determining the capacity of N transport and assimilation and other nitrate responses. We propose that the NLP-NIGT1 cascade is one of critical modulators for nitrate-responsive transcription on the basis of our findings; however, other factors may act to regulate the temporal expression patterns of nitrate-inducible genes including NRT2 . 1 , because the mutated NRT2 . 1 promoter with the disruptions of NIGT1-biding sites was still repressed during nitrate treatment. One of such factors may be the nitrate-induced accumulation of N-metabolites and cytokinin that repress the expression of nitrate-inducible genes, including NRT2 . 1 [25] , [26] , [49] , [51] . Another is degradation of NLPs, because NLPs in the active form were more rapidly degraded, compared with ones in the inactive form (Supplementary Fig. 11 ). Fig. 9 Model for the NIGT1-centred transcriptional cascade. a Model for the transcriptional cascade that modulates nitrate uptake in response to fluctuations in the nitrate condition. Nitrate activates NLP, which directly upregulates both the NRT2 . 1 and NIGT1-clade gene promoters. Thus, NRT2 . 1 expression is initially activated (1) and then repressed by expression of NIGT1 - clade genes (2). Increases in NRT2 . 1 expression lead to enhanced uptake of nitrate as a substrate for nitrate assimilation and also a signal for activating NLP. The expression level of NRT2 . 1 is modulated by the balance of these positive and negative regulatory loops. b Model for the transcriptional cascade that integrates nitrate and P-starvation signalling pathways. When P nutrient (phosphate) is abundant, PHR1 is kept inactive by the SPX–inositol polyphosphate (*) complex. Thus, the nitrate-NLP cascade activates the NRT2 . 1 promoter independently of the PHR1 pathway. Upon P depletion, PHR1 is freed and enhances the expression of NIGT1-clade genes, leading to reductions in both NRT2 . 1 expression and nitrate uptake Full size image Antagonistic regulation by NLPs and NIGT1s may explain not only transient changes in nitrate-inducible expression after nitrate supply but also different expression levels at the steady state under different N concentrations. As reported previously, NRT2 . 1 expression is high at appropriate concentrations of nitrate but is lower at higher concentrations of nitrate [24] , [25] , [26] . This may be partly mediated by N-metabolites [25] , [26] , [49] , but, as the phenomenon is observed even in the presence of ammonium, nitrate itself is a key determinant [31] . When the nitrate concentration is higher than the appropriate concentration range, higher amounts of NIGT1s may accumulate and suppression by NIGT1s may dominate. Consistent with this hypothesis, two NIGT1-binding sites are located in the 150 bp promoter region of the NRT2 . 1 promoter that was previously shown to be involved in both activation under low nitrate conditions and repression under high N conditions [25] . Although the NIGT1-mediated repression appeared to be more evident in the presence of high concentration of nitrate (Supplementary Fig. 5 ), further analyses would be necessary to clarify the role of NIGT1 in the presence of high concentrations of nitrate. Our findings highlight a new mechanism to explain modulations of nitrate response. The presence of conserved NIGT1 sites in the promoters of Arabidopsis NIGT1-clade genes and Os NIGT1 suggests that the NIGT1-mediated regulatory mechanism prevails among various plant species. In fact, the maize homologue of Os NIGT1 (GRMZM2G016370), which was annotated as MYB-like gene, was upregulated by high N supply [52] . Hence, even if nitrate-inducible gene expression is also downregulated by other N metabolite-dependent pathways [25] , [26] , [51] , [53] or degradation of the activated forms of NLPs (Supplementary Fig. 11 ), the NIGT1 pathway would be a useful target for modification of nitrate responses to improve N utilisation and productivity in various crop species. Our findings also uncovered a molecular mechanism for integration of nitrate and P-starvation signalling (Fig. 9b ). Plants require nutrients in appropriate ratios, because deficiency of one particular nutrient may lead to excess accumulation of other nutrients. Similarly, abundance of one nutrient may lead to deficiencies of other nutrients. Such interdependence is exhibited by N and P, both of which are required in abundance for optimal plant growth and are hence found in large quantities in plant fertilisers. P limitation inhibits N uptake in tobacco [40] , barley [38] and maize [39] , and is accompanied by an accumulation of amino acids [40] , [54] , [55] . These phenomena suggest that plants possess regulatory mechanisms to coordinate the uptake and utilisation of nutrients to maintain metabolic homeostasis. NLA ubiquitin E3 ligase was shown to mitigate nitrate limitation-induced P accumulation [56] through the degradation of PHT1 phosphate transporters [57] , and phenotypic analysis implicated NIGT1s in integration of N and P signals [36] . However, elucidation of N and P mechanisms coordinating N and P metabolism remained largely elusive. In the model based on our findings (Fig. 9b ), under the P-sufficient condition, PHR1 interacts with SPXs, P sensor proteins, and inhibitors for PHR1 [58] , [59] , and NIGT1 - clade genes are not activated. Under P-starved conditions, PHR1 is released from SPXs and promotes expression of NIGT1-clade genes. Therefore, nitrate uptake is partly decreased by P-starvation via the PHR1-NIGT1-NRT2.1 pathway. The inhibition of N uptake lowers the rate of anabolism and thus decreases the demand for P. Hence, the regulation of N uptake by the PHR1-NIGT1 pathway may be a strategy to adapt to P deficiency, although other mechanisms, such as general reductions in biosynthesis, likely contribute to reductions in N uptake under P-deficient conditions. NIGT1 - clade gene expression was more strongly induced by nitrate signalling than by P-starvation signalling (Figs. 2 , 7 ). Thus, NIGT1s primarily act as modulators for nitrate response, and the role in P-starvation signalling is presumably ancillary. This is consistent with fundamental regulation of nitrate uptake by N-nutrient condition and secondary regulation by P availability. Unexplained observations, such as the reduction of NRT2 . 1 promoter activity in the absence of NIGT1-binding, indicate that the model shown in Fig. 9b requires refinement by additional analyses and incorporation of other factors. However, the key finding of the current study is that two independent transcriptional cascades for nitrate and P-starvation signalling are integrated via expression control of NIGT1-clade genes. Phenotypic analysis revealed that constitutive overexpression of NIGT1 . 1 severely affected growth, leading to smaller shoots and shorter primary roots, irrespective of the nitrate concentration (Supplementary Fig. 12a, b ). Conversely, quadruple nigt1 mutants displayed slight reductions in total lateral root length, although shoot fresh weight and primary root length were similar to those of the wild type (Supplementary Fig. 12 ). Previous phenotypic analysis indicated that NIGT1 . 3 and NIGT1 . 4 were involved in primary root shortening under P-deficient conditions [35] , [36] and NIGT1 . 2 was involved in the promotion of lateral root growth [37] . These observed phenotypes might suggest differences in expression patterns and/or target genes of different NIGT1s. Although NLP7 and NIGT1-clade genes appear to be expressed in most cell types in roots, the cells where NIGT1 . 1 and NIGT1 . 2 are predominantly expressed appear to be are somewhat different from the cells where NIGT1 . 3 and NIGT1 . 4 expression are predominant (Supplementary Fig. 6b ). Detailed analyses including cell-type specificity of the expression of NIGT1-clade genes and NIGT1 protein stability [36] would allow our model to be refined to explain the observed phenotypes. Plant materials Arabidopsis ecotype Columbia (Col) was used as the wild type. T-DNA insertion lines GABI_267G03 [60] ( nigt1 . 1-1 ), SALK_044835C ( nigt1 . 2-1 / hho2-1 ) [37] , SALK_070096 ( nigt1 . 2-2 / hho2-2 ) [37] , SAIL_28_D03 ( nigt1 . 3 / hho1-1 ) [36] , WiscDsLoxHS231_10C ( nigt1 . 3 − 2 ), SALK_067074 ( nigt1 . 4-1/hrs1-1 ) [35] , SALK_067629C ( phr1 ) [37] , SALK_036557 ( nlp6 ) [61] , SALK_026134 ( nlp7-1 ) [11] and SAIL_731_B09 ( phl1 ) [42] were obtained from the Arabidopsis Biological Resource Center or Max-Planck Institute (Supplementary Fig. 8 ). The nigt1 quadruple, nlp6 nlp7-1 double and phr1 phl1 double mutants were generated by crossing T-DNA lines and selecting plants homozygous for all T-DNA alleles using PCR-based genotyping. 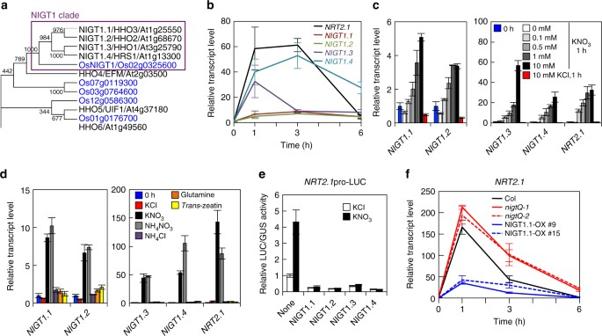Fig. 2 NIGT1 proteins redundantly regulateNRT2.1expression.aPhylogenic analysis ofArabidopsisand rice NIGT1/HHO proteins.Arabidopsisand rice proteins are shown in black and blue, respectively. Numbers indicate bootstrap values of 1000 iterations.bTime-dependent expression patterns of NIGT1-clade genes after 10 mM KNO3supply.cConcentration-dependent induction by nitrate. RNA was prepared from ammonium-grown seedlings before treatment and after treatment with 0, 0.1, 0.5, 1 and 10 mM KNO3for 1 h. A 10 mM KCl treatment was used as a control.dNitrate-specific induction of NIGT1-clade genes. Ammonium-grown seedlings were treated for 1 h with 10 mM of each chemical, except fortrans-zeatin (5 µM).eRepression of theNRT2.1promoter by NIGT1 proteins. Protoplasts co-transfected with NIGT1 expression vectors or the empty vector (none) together with the reporter plasmid containing theLUCgene under the control of theNRT2.1promoter were incubated in the presence of 1 mM KCl or KNO3. LUC activity was normalised to GUS activity from the co-transfected UBQ10-GUS plasmid. Data are means ± s.d. of three biological replicates.fTranscript levels ofNRT2.1in thenigt1quadruple mutants (Q-1andQ-2) and NIGT1.1-OX plants after 10 mM KNO3supply. Values are normalised to those ofUBQ10, and are means of biological triplicates ± s.d. (b,c,d,f) Primers used for genotyping are listed in Supplementary Table 2 . The transgenic lines expressing the chimeric repressor form of NLP6 (NLP6-SUPRD) were described previously [8] . The NIGT1.2-GFP-OX line that was generated by transformation of Col plants [46] expresses NIGT1.2-GFP fusion protein under the control of the 35S promoter. Plant growth conditions Seeds were stratified at 4 °C for 3−4 days. Plants were grown at 23 °C with continuous illumination (60 µmol m −2 s −1 ) under a variety of nutrient conditions denoted for each experiment. Dark growth treatments are noted in the relevant experimental procedures. Agar media comprised 0.5× Murashige and Skoog salts [62] (1/2MS) buffered with 0.5 g l −1 MES-KOH (pH 5.7) and solidified with 0.8% agar. Liquid media comprised 0.1× MS salts (1/10MS) buffered with 0.1 g l −1 MES-KOH (pH 5.7). Supplementation with sucrose or K + (as K 2 SO 4 ) is indicated where relevant. When modification of N source or concentration was required, KNO 3 and NH 4 NO 3 in MS salts were omitted or replaced with the indicated N source. For P-starvation treatment, KH 2 PO 4 was omitted and the concentration of FeSO 4 was lowered to 0.4 µM to avoid possible detrimental effects of excess iron [63] . Plasmid construction Reporter plasmids for transient assays, pNRT2.1p-LUC and pNIGT1pro-LUC, harboured the NRT2 . 1 or NIGT1 gene promoter upstream of the LUC gene. To construct plasmids, a 1.3 kb NRT2 . 1 promoter fragment and 1 kb NIGT1 promoter fragments were amplified from genomic DNA by PCR and cloned between the Hin dIII and Nco I sites of pJD301 [64] . NRT2 . 1 and NIGT1 . 1 promoter fragments carrying mutations were produced by the overlapping PCR method and similarly cloned into pJD301 to generate (mut1)-LUC, (mut2)-LUC, (mut3)-LUC, (mut1+2)-LUC, (mut1+2+3)-LUC, (D1mut)-LUC, (P1mut)-LUC, (P2mut)-LUC, (P1P2mut)-LUC, and (D1P1P2mut)-LUC plasmids and pNIGT1pro-LUC-related plasmids. The effector plasmids for the transient expression of MYC-tagged LBD37, NIGT1.1-1.4, and PHR1 in protoplasts were generated by replacing the cDNA of EIN3 in p35S-C4PPDK-EIN 3 − MYC [65] with LBD37 , NIGT1 . 1-1 . 4 , or PHR1 cDNA obtained by RT-PCR. The NLP7 expression plasmid and the internal control plasmid pUBQ10-GUS were described previously [8] . The pET32-NIGT1.1(DBD) plasmid for production of recombinant NIGT1.1 protein in E . coli was generated by insertion of a DNA fragment encoding the GARP domain of NIGT1.1 between the Nco I and Xho I sites of pET32. The pET32-based plasmid for the production of recombinant NLP7(DBD) was described previously [8] . A binary plasmid for overexpression of NIGT1 . 1 tagged with six copies of the MYC epitope-encoding sequence was generated by replacing the 35SΩ promoter sequence and NLP6 cDNA in pCB302HYG-35SΩ-NLP6-MYC [10] with the 1.5 kb sequence of the UBQ10 promoter and NIGT1 . 1 cDNA. A binary plasmid for expression of PHR1 tagged with six copies of the MYC epitope-tag was generated by replacing NLP6 cDNA in pCB302HYG-35SΩ-NLP6-MYC [10] with PHR1 cDNA. Binary plasmids for the expression of LUC under the control of wild-type or mutated NRT2 . 1 promoters were generated by replacing the 35SΩ sequence of pCB302-35SΩ-LUC [66] with the NRT2 . 1 promoter fragments of NRT2 . 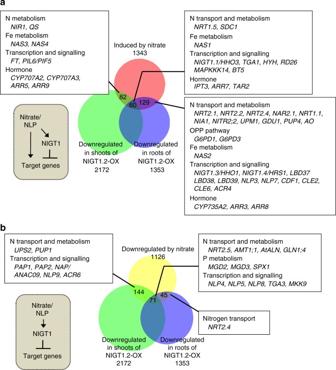Fig. 3 Nitrate-responsive and NIGT1-regulated genes.aA Venn diagrams showing an overlap between genes upregulated by nitrate after 30 min or 3 h and genes downregulated in NIGT1.2-overexpressing plants.bA Venn diagram showing an overlap between genes downregulated by nitrate after 30 min or 3 h and downregulated in NIGT1.2-overexpressing plants. Numbers of genes are shown. Note thatNRT2.4was upregulated at 30 min after nitrate treatment but downregulated at 3 h 1 p-LUC and (mut1+2)-LUC plasmids. All PCR products were verified by DNA sequencing. Primers are listed in Supplementary Table 2 . Co-transfection assay Arabidopsis Col seeds on a urethane sponge wetted with 1/10MS solution were incubated under continuous illumination for 1 day and subsequently in the dark for 2 days. Etiolated seedlings were then hydroponically grown with 1/10MS solution in the light for 17 days and then with N-free 1/10MS solution supplemented with 0.5 mM K 2 SO 4 for an additional 3 days for N-starvation treatment. Preparation of mesophyll protoplasts and co-transfection of plasmids into protoplasts were performed as described in Yoo et al. [67] . Co-transfections with 2×10 4 protoplasts were carried out with 20 µg total of plasmids (6 µg of the reporter plasmid, 12 µg of the effector plasmid, and 2 µg of pUBQ10-GUS). For simultaneous introduction of two effector plasmids at different ratios, 2.6 µg of the reporter plasmid, 5.2 µg (for ratio: 1) or 10.4 µg (for ratio: 2) of the effector plasmids, and 2 µg of pUBQ10-GUS was used. Total plasmid amounts for each transfection were adjusted to 20 µg with the empty (none) plasmid. Transfected protoplasts were incubated in WI solution [67] in the dark overnight. For nitrate treatment, transfection of N-starved protoplasts was similarly performed but with 4×10 4 protoplasts and 40 µg of plasmids. One half each of the transfected protoplasts was incubated in WI solution supplemented with KCl or KNO 3 in the dark overnight. The final concentration of KCl and KNO 3 in WI solution was noted in the relevant figure legends. LUC and β-glucuronidase (GUS) assays were performed with the Luciferase Assay System (Promega) and 4-methylumbelliferyl-β- d -glucuronide, respectively. LUC activities were normalised to GUS activities produced by the reference plasmid pUBQ10-GUS. Triplicate biological samples were analysed with consistent results. Co-transfection assays were performed at least two times with similar results. EMSA DNA probes were prepared using two rounds of PCR. The first round of PCR was performed with NRT2.1p-LUC, (mut1)-LUC, (mut2)-LUC or (mut3)-LUC plasmids as template and specific primer pairs. Reverse primers for NIGT1-binding assays also carried the M13 reverse primer sequence, and the primers for NLP7-binding assays contained OligoY or Z sequence (Supplementary Table 2 ). After purification of PCR products through electrophoresis with an acrylamide gel, the second round of PCR was performed with the purified PCR product as a template, using the same forward primer and a biotin-labelled M13 primer (for NIGT1-binding assays) or biotin-labelled OligoY and OligoZ (for NLP7-binding assays). The secondary PCR products were purified using the Wizard ® SV Gel and PCR Clean-Up System (Promega) and used as biotin-labelled probes. The OsNIGT1 probe used as a positive control was similarly produced by two rounds of PCR. This probe corresponded to a region of the Os NIGT1 promoter (−251 to −95 relative to the translation start codon) and contained one conserved and one nonconserved NIGT1-binding sequence [17] . Recombinant Trx- and His-tagged NIGT1.1(DBD) and NLP7(DBD) proteins were produced in E. coli BL21(DE3) cells transformed with the pET32-NIGT1.1(DBD) and pET32-NLP7(DBD) plasmids, respectively, and purified using Complete His-tag Purification Resin (Roche). Binding of the recombinant protein (25–50 ng) to DNA probes (2.5–5 ng) was carried out in a reaction mixture containing 0.5 µg of poly[d(I-C)], 20 mM HEPES-KOH (pH 7.6), 3 mM MgCl 2 , 30 mM KCl, 20 mM NaCl, 2 mM dithiothreitol, 0.5 mM EDTA (pH 8.0), 10% glycerol, and 0.1× EDTA-free Complete (Roche). Electrophoresis was performed with native 5% polyacrylamide gels in 0.5× TBE. Probe DNAs transferred onto the positively charged nylon membranes (Biodyne B, PALL) were detected with streptavidin-horseradish peroxidase (Pierce). The results were verified by two independent experiments (Pierce). RT-qPCR analysis RT-qPCR analysis of nitrate induction was performed with Arabidopsis seedlings that were grown in N-free 1/10MS solution supplemented with 0.5 mM ammonium succinate as a N source and 0.5% sucrose for 5 days. KNO 3 or other N compounds were supplied to induce related gene expression, and seedlings were collected after 1, 3 or 6 h. For RT-qPCR analysis with P-starved plants, Col and phr1 phl1 seeds were germinated on a urethane sponge wetted with N-free 1/10MS medium supplemented with 0.2 mM KNO 3 , and seedlings were grown under illumination for 1 day and subsequently in the dark for 2 days. Etiolated seedlings were then hydroponically grown with the same medium for 13 days. 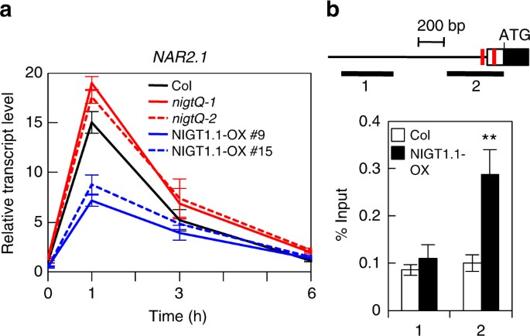Fig. 4 Repression ofNAR2.1by NIGT1s.aTime-dependent expression ofNAR2.1inArabidopsisCol,nigt1quadruple mutants (Q-1andQ-2), and two NIGT1.1-OX lines (#9 and #15). Seedlings were harvested at the indicated time points after supply of 10 mM KNO3. Values are normalised with expression levels ofUBQ10, and means of biological triplicates ± s.d. are shown.bBinding of NIGT1.1 to theNAR2.1promoter in vivo. ChIP analysis was carried out with Col and NIGT1.1-OX seedlings. Two different regions of theNAR2.1promoter that contained or did not contain putative NIGT1-recognition sequences (red bars) were amplified from immunoprecipitated DNA by PCR. Data are means of four biological replicates with s.d. **p< 0.01 by one-tailedt-test compared with corresponding values obtained with Col seedlings Plants were then transferred to the same fresh medium or fresh medium without P and grown for 5 days. Total RNA from seedlings was prepared with ISOGEN reagent (NIPPONGENE, Tokyo, Japan) or with an ISOSPIN plant RNA kit (NIPPONGENE). RT reactions were performed using SuperScriptII reverse transcriptase (Thermo Fisher Scientific), and qPCR was performed with a StepOne Plus™ Real Time PCR System (Applied Biosystems) and the KAPA SYBR Fast qPCR Kit (KAPA Biosystems). Triplicate biological samples were analysed with consistent results, and the results were verified by two independent experiments. Generation of transgenic plants Transformation of Arabidopsis was performed by the floral dip method using Agrobacterium strain GV3101 (pMP90) [68] . Lines that exhibited a segregation of 3:1 for glufosinate ammonium or hygromycin B resistance at the T 2 generation were selected, and T3 progenies of the lines that were homozygous for the introduced gene were used for all analyses in this study. ChIP assay For ChIP analysis with NIGT1.1-OX #9 plants, seedlings were grown for 10 days on agar plates that contained 1/2MS salts, 3 mM MES-KOH (pH 5.8), 0.5% sucrose and 0.8% agar. For ChIP analysis with PHR1-OX plants, etiolated seedlings were generated by cultivation for 1 day under continuous illumination and then 2 days in the dark. Plants were then hydroponically grown with 1/10MS solution for 13 days and then 1/10MS solution without P for 5 days. ChIP was performed using the protocol of Saleh et al. [69] with slight modifications. In brief, after cross-linking proteins to DNA and isolation and lysis of nuclei, DNA sonication was performed with a BIORUPTOR ® II (COSMO BIO CO., LTD, Tokyo, Japan) at high mode, 10× 30 s, with 30-s intervals. Immunoprecipitation was carried out with Protein A or G-agarose beads (Roche) conjugated to 5 µg of anti-MYC antibody (clone 9E10, Millipore #05-419) overnight at 4 °C. DNA recovered from agarose beads was purified using a DNeasy Plant Mini Kit (Qiagen). qPCR was performed with a StepOne Plus™ Real Time PCR System (Applied Biosystems) and the KAPA SYBR Fast qPCR Kit (KAPA Biosystems). Three or four biological samples were analysed with consistent results. Imaging of LUC activity in vivo For in vivo LUC imaging of NH 4 NO 3 -treated plants harbouring the NRT2.1p-LUC and (mut1+2)-LUC construct, we introduced these constructs into the wild-type Arabidopsis (Col). 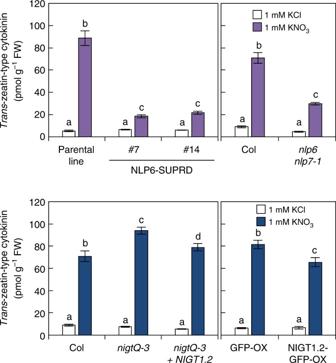Fig. 5 NLP and NIGT1 activity affects tZ-type cytokinin content. Cytokinin contents in the seedlings treated with 1 mM KNO3or KCl for 24 h were measured. The cytokinin contents in two NLP6-SUPRD lines were compared with those in its parental line (4xNRE-35Smin-GUS)21, and the cytokinin contents in thenlp6 nlp7-1mutant, thenigt1quadruple mutant (nigtQ-3), and the complementation line ofnigtQ-3, which was produced by expression ofNIGT1.2, were compared with those in Col seedlings. The cytokinin contents in the NIGT1 overexpressor (NIGT1.2-GFP-OX), which was produced by the overexpression of NIGT1.2 fused to GFP, were compared with those in the GFP overexpressor line (GFP-OX). Values are mean ± s.d. (n= 4~5). Different letters denote significant difference by Tukey’s HSD (p< 0.05) Five T3 seedlings of each resultant transgenic line were grown in 3 ml of N-free 1/10MS medium supplemented with 2 mM KNO 3 and 0.5% sucrose in one well of six-well plates for 5 days. Ammonium nitrate solution was then added into the medium at a final concentration of 10 mM, and seedlings were incubated for 24 h. An equal amount of water was added to control seedlings. For analysing effects of different concentrations of nitrate, three seedlings were grown in 5 ml of N-free 1/10MS medium supplemented with indicated concentrations of KNO 3 and 0.5% sucrose in one well of six-well plates for 6 days. For in vivo LUC imaging of P-starved NRT2 . 1 p-LUC and (mut1+2)-LUC plants, seedlings were grown in N-free 1/10MS medium supplemented with 1 mM KNO 3 and 0.5% sucrose for 5 days. The medium was then changed to N-free 1/10MS medium supplemented with 0.5 mM KNO 3 , 0.25 mM K 2 SO 4 and 0.5% sucrose, and seedlings were incubated for 1 day. Seedlings were then grown with 1/10MS-based medium with or without P. Nutrient solutions were then changed daily. 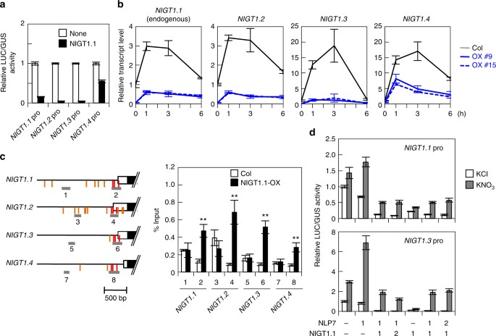Fig. 6 Autoregulation of NIGT1-clade genes.aRepression of NIGT1-clade gene promoters by NIGT1.1. A reporter plasmid that contained theLUCgene under the control of anNIGT1promoter was co-transfected in protoplasts alongside the NIGT1.1 expression vector and the UBQ10-GUS reference plasmid. LUC activity was normalised with GUS activity. Data are means ± s.d. of three biological replicates.bReduced expression of endogenousNIGT1.1as well asNIGT1.2,NIGT1.3andNIGT1.4in NIGT1.1-OX lines. Ammonium-grownArabidopsisCol and NIGT1.1-OX seedlings were treated with 10 mM KNO3for the indicated periods and used for RT-qPCR analysis. Values are normalised toUBQ10expression levels, and means of biological triplicates with s.d. are shown.cBinding of NIGT1.1 to theNIGT1gene promoters in vivo. ChIP analysis was performed with Col and NIGT1.1-OX seedlings. Two different promoter regions were amplified from immunoprecipitated DNA. Data are means of four biological replicates with s.d. **p< 0.01 by one-tailedttest compared with corresponding values obtained with Col seedlings. Positions of the conserved and nonconserved putative NIGT1-binding sites are shown by vertical red and orange lines, respectively.dAntagonistic regulation of NIGT1-clade gene promoters by NLP7 and NIGT1.1. Expression vectors for NLP7 and NIGT1.1 were co-transfected into protoplasts at different ratios, together with a reporter plasmid containing theLUCgene under the control of theNIGT1.1orNIGT1.3promoter. Transfected protoplasts were incubated in the presence of 10 mM KCl or KNO3. LUC activity was normalised with GUS activity, and relative LUC activities are means ± s.d. of three biological replicates For in vivo imaging of LUC activity, luciferin potassium salt (Wako, Osaka, Japan) was added to the medium at a final concentration of 1 mM. 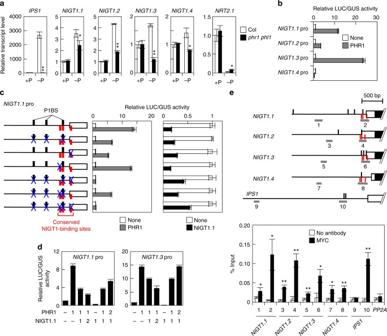Fig. 7 PHR1-dependent activation of NIGT1-clade genes.aEffects of P starvation on the expression of NIGT1-clade genes andNRT2.1in roots ofArabidopsisCol andphr1 phl1double mutant. Roots ofArabidopsisplants that were grown hydroponically under P-sufficient (+P) or P-starved (−P) conditions for 5 days were used for RT-qPCR analysis.IPS1is a positive control for P starvation. Values are normalised with expression levels ofPEX4, and means of biological triplicates with s.d. are shown. *p< 0.05, **p< 0.01 by two-tailedt-test compared with corresponding Col values.bTransactivation of NIGT1 promoters by PHR1. A reporter plasmid containing 1 kb promoter fragments of NIGT1-clade genes fused to theLUCgene was co-transfected into protoplasts with the PHR1 expression vector or an empty vector (none) and the UBQ10-GUS plasmid.cIdentification of sites mediating PHR1 regulation and autoregulation in theNIGT1.1promoter. Transactivation of wild-type and mutatedNIGT1.1promoters by PHR1 and repression by NIGT1.1 were analysed by co-transfection assays. The horizontal line indicates the 1 kbNIGT1.1promoter. Vertical black and red lines indicate the P1BS sequences and the conserved NIGT1 sites, respectively. Mutated sites are indicated with blue X.dCompetitive regulation of the NIGT1-clade gene promoters by PHR1 and NIGT1. Expression vectors for PHR1 and NIGT1.1 were co-transfected into protoplasts at different ratios, together with theLUCreporter gene under the control of theNIGT1.1orNIGT1.3promoter. Inb−d, relative LUC activity is given as mean ± s.d. of three biological replicates.eBinding of PHR1 to the NIGT1-clade gene promoters in vivo. Two different regions from each NIGT1-clade gene promoter were amplified in a ChIP assay of transgenic plants expressing MYC-tagged PHR1 cultured under the P-starved condition. TheIPS1promoter is a known target of PHR1 and is used as a positive control, andPP2Ais a negative control. Data are means of three biological samples and shown with s.d. *p< 0.05, **p< 0.01 by one-tailed pairedt-test compared with corresponding control (no antibody) values After incubating in the dark for 10 min, luminescence from the seedlings was detected using an Amersham Imager 600 (GE Healthcare) with 60 min exposure. The obtained 16 bit images were converted to pseudo-colour using ImageJ software (NIH, USA). Genome-wide survey of genes under the control of NIGT1s Arabidopsis genes regulated by nitrate were identified using published data [7] . Nitrate-upregulated genes were those that met both of the following criteria: (1) the expression level in KNO 3 -treated samples was more than twofold higher than expression in control (no treatment) samples; and (2) the expression level in KNO 3 -treated samples was more than twofold higher than expression in KCl-treated samples. Nitrate-downregulated genes were those that met both of the following criteria: (1) the expression level was more than twofold lower in KNO 3 -treated samples than in control (no treatment) samples; and (2) the expression level in KNO 3 -treated samples was more than twofold lower than expression in KCl-treated samples. Genes downregulated by NIGT1.2-OX were described in Kiba et al. [46] (accession number GSE100903 in Gene Expression Omnibus). Venn diagrams with numbers of selected genes were generated by BioVenn . Quantification of cytokinin Seedlings were grown in N-free 1/2MS liquid medium supplemented with 1% sucrose at 22 ℃ under continuous light with rotation (120 rpm) for 4 days and treated with 1 mM KCl or 1 mM KNO 3 for 12 h before harvest. Extraction and determination of cytokinin was performed with the same system constructed in Kojima et al. [70] In brief, the extract obtained from about 100 mg of seedlings with the extraction solvent (methanol:formic acid:water = 15:1:4) was mixed with internal standards labelled with stable isotopes and loaded onto an Oasis MCX 96-Well Plate 30 mg (Waters) equilibrated with 1 M formic acid. After washing with 1 M formic acid and then with methanol, cytokinin nucleotides were eluted with 0.35 M ammonia, and then cytokinin nucleobases were eluted with 0.35 M ammonia in 60% (v/v) methanol. The eluate containing cytokinin nucleotides was reconstituted with 0.84 ml of 0.1 M N -cyclohexyl-2-aminoethanesulfonic acid-NaOH (pH 9.8) and treated with alkaline phosphatase (17 µl of 1 U μl −1 , Oriental Yeast Co. Ltd., Tokyo, Japan) for 1 h at 37 °C. After the treatment, 93 μl of 10× Tris-buffered saline and 46 μl of 1 M HCl were added into the reaction mixture. Then, the mixture was desalted by passing through a water-equilibrated Oasis HLB 96-Well Plate 30 mg (Waters), and cytokinin nucleotides were eluted with methanol. After evaporation of methanol, cytokinin nucleotides were dissolved in 50 μl of 0.1% acetic acid and were subjected to ultra-performance liquid chromatography coupled with a tandem quadrupole mass spectrometer equipped with an electrospray interface (UPLC-ESI-qMS/MS; AQUITY UPLC™ System/Quattro Ultima Pt, Waters) analysis with an ODS column (AQUITY UPLC BEH C 18, Waters). On the other hand, solvents of the eluate containing cytokinin nucleobases were evaporated, and cytokinin nucleobases were dissolved in 50 μl of 0.1% acetic acid and subjected to UPLC-ESI-qMS/MS analysis. Data were processed by the MassLynx™ software with QuanLynx™ (Waters). 15 NO 3 − uptake Etiolated seedlings generated by growth under illumination for 1 day and in the dark for 2 days were then hydroponically grown with 1/10MS solution in the light for 13 days. Plants were then grown with 1/10MS solution with or without P for 5 days. Plant roots were submerged in 0.1 mM CaSO 4 for 1 min and then medium containing 0.2 mM K 15 NO 3 for 5 min. After washing in 0.1 mM CaSO 4 for 1 min [28] , roots were collected and dried. N content and 15 N ratio were analysed by SI Science Co. Ltd. (Tokyo, Japan). Five biological replicates were analysed with consistent results. Immunoblot analysis Seedlings of the transgenic lines expressing MYC-tagged NLP7 [10] were grown in N-free 1/10MS solution supplemented with 0.5 mM ammonium succinate (Nitrogen-free 1/10 MS salts, 0.1 g l −1 MES-KOH (pH 5.7), 0.5% sucrose, 0.5 mM ammonium succinate) for 4 days and the solution was then changed to the same fresh solution but containing 10 mM KCl or KNO 3 . Seedlings were collected 0, 0.5, 1, 3, 6 and 24 h after the change of the solution. The seedlings were weighed, frozen in liquid nitrogen and ground using a Multibeads Shocker (Yasui Kikai, Osaka, Japan). The ground samples were suspended in 10 volume of 1× Laemmli sample buffer supplemented with EDTA-free protease inhibitor cocktail (Roche) and heated at 95 °C for 30 s. Samples were then subjected to SDS-PAGE and immunoblotting with anti-MYC (Millipore, 05-419; 1:1000) and anti-Histone H3 (Abcam, ab1791; 1:5000) antibodies. Phenotypic analysis Seeds of Col, NIGT1 overexpressors and nigt1 quadruple mutants were germinated on 1/2MS plates (1/2MS salts, 0.5 g l −1 MES-KOH (pH 5.7), 1% sucrose and 0.8% agar). Seedlings were grown on plates for 3 days and then transferred to vertically placed test plates (N-free 1/2MS salts, 0.5 g l −1 MES-KOH (pH 5.7), 1% sucrose and 0.8% agar) supplemented with the indicated concentrations of KNO 3 and NH 4 NO 3 and grown for 6 days. The upper 2 cm part of the agar medium was removed from test plates to avoid contact of shoots with the medium. Images of agar plates were taken using an Amersham Imager 600 (GE Healthcare), and root lengths were measured using ImageJ software (NIH, USA). The results were verified by two independent experiments. 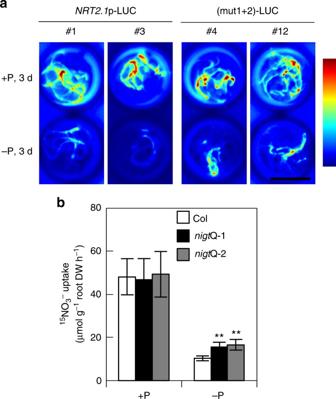Fig. 8 The PHR1-NIGT1 cascade modulates nitrate uptake.aNIGT1-binding site-mediated P-starvation response ofNRT2.1promoter activity. TransgenicArabidopsisseedlings harbouring theLUCgene under the control of the wild-type or (mut1+2) mutantNRT2.1promoter were grown under P-sufficient (+P) or P-starved (−P) conditions for 3 days and then treated with 1 mM luciferin. Images of LUC activity in living seedlings were captured in two independent transgenic lines. Scale bar, 1 cm.bNitrate uptake activity ofnigt1quadruple mutants (Q-1andQ-2) during P starvation.15NO3−uptake byArabidopsisCol and mutant seedlings grown hydroponically under P-sufficient (+P) or P-starved (−P) conditions for 5 days was measured at 0.2 mM K15NO3. Values are means of five biological replicates ± s.d. **p< 0.01 by two-tailedt-test 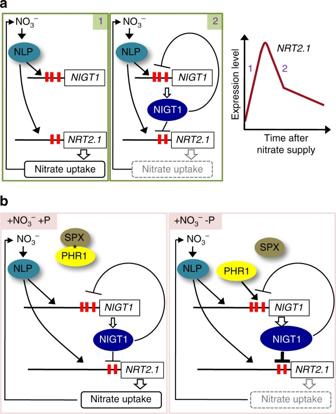Fig. 9 Model for the NIGT1-centred transcriptional cascade.aModel for the transcriptional cascade that modulates nitrate uptake in response to fluctuations in the nitrate condition. Nitrate activates NLP, which directly upregulates both theNRT2.1and NIGT1-clade gene promoters. Thus,NRT2.1expression is initially activated (1) and then repressed by expression of NIGT1-clade genes (2). Increases inNRT2.1expression lead to enhanced uptake of nitrate as a substrate for nitrate assimilation and also a signal for activating NLP. The expression level ofNRT2.1is modulated by the balance of these positive and negative regulatory loops.bModel for the transcriptional cascade that integrates nitrate and P-starvation signalling pathways. When P nutrient (phosphate) is abundant, PHR1 is kept inactive by the SPX–inositol polyphosphate (*) complex. Thus, the nitrate-NLP cascade activates theNRT2.1promoter independently of the PHR1 pathway. Upon P depletion, PHR1 is freed and enhances the expression of NIGT1-clade genes, leading to reductions in bothNRT2.1expression and nitrate uptake Data availability The datasets generated and/or analysed during the current study are available from the corresponding author on reasonable request.